Sculpting carbon bonds for allotropic transformation through solid-state re-engineering of –sp2carbon Carbon forms one of nature’s strongest chemical bonds; its allotropes having provided some of the most exciting scientific discoveries in recent times. The possibility of inter-allotropic transformations/hybridization of carbon is hence a topic of immense fundamental and technological interest. Such modifications usually require extreme conditions (high temperature, pressure and/or high-energy irradiations), and are usually not well controlled. Here we demonstrate inter-allotropic transformations/hybridizations of specific types that appear uniformly across large-area carbon networks, using moderate alternating voltage pulses. By controlling the pulse magnitude, small-diameter single-walled carbon nanotubes can be transformed predominantly into larger-diameter single-walled carbon nanotubes, multi-walled carbon nanotubes of different morphologies, multi-layered graphene nanoribbons or structures with sp 3 bonds. This re-engineering of carbon bonds evolves via a coalescence-induced reconfiguration of sp 2 hybridization, terminates with negligible introduction of defects and demonstrates remarkable reproducibility. This reflects a potential step forward for large-scale engineering of nanocarbon allotropes and their junctions. Carbon nanotubes (CNTs) have attracted considerable interest over the past two decades as they offer a unique combination of physical properties and chemical stability [1] . Particularly, CNT networks are anticipated to be used in broader applications, such as reinforcements for lightweight and high performance composites, multifunctional membranes, electronics and electrodes for energy storage devices [2] , [3] , [4] , [5] , [6] . However, most assembled CNT networks are mainly based on weak van der Waals interactions between the CNTs in CNT arrays [7] . As a result, the reported experimental mechanical strength, and electrical and thermal conductivities are several orders of magnitude lower than theoretical predictions due to a lower mechanical pulling resistance between nanotubes, and a higher electron and phonon scattering at these ‘unconnected’ junctions. Recently, there has been significant success and a growing interest in transforming these van der Waals interactions into covalently bonded molecular junctions [8] , [9] , [10] , [11] , [12] , [13] , [14] , [15] , [16] , [17] , [18] , [19] , [20] , [21] , [22] , [23] , [24] , [25] , [26] , [27] , [28] , [29] . For example, electron [11] , [19] , [20] , [21] and ion [11] irradiation as well as electrical current sources [23] , [24] , [25] , [26] , [27] have been used to modify the structure and morphology of nanocarbons. However, these rearrangement studies were carried out only for local changes of junctions in a few individual nanotubes [11] , [12] , [13] , [14] , [15] , [16] , [17] , [18] , [19] , [20] , [21] , [25] and by the destruction of carbon layers on electrical breakdown [23] , [26] , [27] . Furthermore, the reported reconstruction methods require high to extremely high temperature (750–2,200 °C) conditions [20] , [22] , [28] , making them power-intensive, and incompatible with various scalable processes. Therefore, developing a fast and scalable method for reproducibly creating particular types of covalently bonded C–C junctions and sp 2 molecular structures in nanocarbon networks that result in repeatable physical properties is still a fundamental challenge. Here we report a method for constructing sp 2 inter-nanotube junctions and desired allotropic structures by applying controlled alternating voltage pulses across single-walled carbon nanotube (SWCNT) networks. Transformations across entire networks (electrode to electrode) were characterized point-by-point with Raman spectroscopy and were also visually inspected using transmission electron microscopy (TEM) before and after the voltage pulse cycling was completed. Our transformation process has several interesting features. First, by controlling the electrical parameters, such as the amplitude, the number of cycles and the duty cycle of an alternating voltage pulse, nearly the entire Raman and TEM-inspected regions of SWCNT networks were found to be transformed uniformly and reproducibly, mostly into either larger diameter SWCNTs, multi-walled carbon nanotubes (MWCNTs) or multi-layered graphene nanoribbons (MGNRs). Second, the new nanocarbon network retains its sp 2 covalent bonds and seamless structures, without increasing structural defects after the transformational process is completed. Third, the method is facile, easily scalable and extendible into 2–3 dimensional [29] and multiscale (nano- to macro-scale) applications. I – V characterization and alternating voltage pulses Highly organized SWCNT micronetworks containing about (2±0.5) × 10 4 CNTs per μm 2 were assembled by using a template-guided fluidic assembly process [30] , [31] , [32] and attached with electrodes for electrical treatment. Particularly for TEM observation, well-defined SWCNT microlines (see Method section) were directly assembled on specially designed TEM grids where micro-windows were located between built-in micro-heaters for external heating. 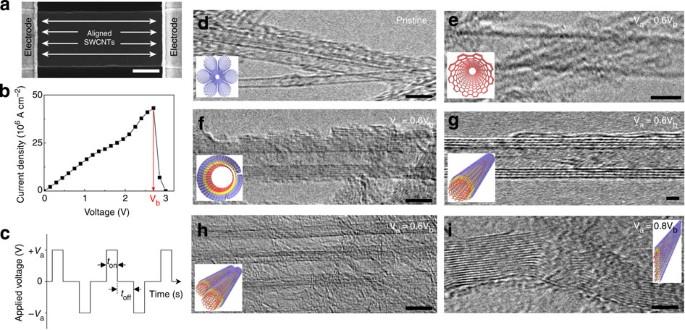Figure 1: Pulsed-alternating-voltage induced allotropic transformation of SWCNTs. (a) SEM image of an assembled SWCNT network integrated with electrodes fabricated on a specially designed TEM grid (seeSupplementary Fig. 1a). A scale bar is 500 nm. (b) TypicalI–Vcharacteristics of a pristine SWCNT network device showing breakdown behaviour beyond the voltage,Vb=2.7 V, corresponding to a maximum current density of about 4.3 × 107A cm−2. (c) Time-dependent alternating voltage pulses that were used to obtain the described transformation of the SWCNT arrays.Va,tonandtoffindicate applied voltage amplitude, and voltage ON and OFF durations, respectively. (d) Typical TEM image of the SWCNTs in the array before the voltage cycling was initiated. (e–i) Typical morphologies of nanocarbon structures obtained after the voltage pulse cycling was completed. In each case,Vais presented in unitsVb. The typical carbon morphologies obtained after cycling 3,000 times atVa=0.6Vbare (e) SWCNTs with a larger diameter, (f) multi-walled tubular structures with several incomplete sp2walls, (g) well-formed MWCNTs and (h) bundles of MWCNTs. (i) MGNRs were obtained typically after the network was subjected to 3,000 cycles ofVa=0.8Vb. Scale bars in (d–i) are all 5 nm. Figure 1a shows the scanning electron microscopy (SEM) image of an assembled SWCNT network microline between two electrodes. Initial I – V characterization was performed to find the maximum current density ( J b ) and the breakdown voltage ( V b ) of assembled SWCNT networks ( Fig. 1b ) under vacuum. Typically, the CNT arrays assembled on the TEM windows ( Supplementary Fig. 1a,b ) failed at current densities of a few tens of 10 6 A cm −2 corresponding to values of 2.5 V< V b <3 V. Figure 1c schematically represents the time-dependent alternating voltage pulses applied on the SWCNT devices. To initiate molecular junction formation and structural evolution in the SWCNT networks, the electrical polarity was switched periodically (typically at 1 Hz for 3,000 cycles) for several applied voltage amplitudes ( V a , Fig. 1c ) ranging from 0.4 V b to 0.8 V b , where the I – V curves turn slightly nonlinear ( Fig. 1b ) because of increased electron–phonon scattering and structural changes [33] . The source-on-time ( t on in Fig. 1c ) for each V a was also varied to obtain the most effective transformation conditions in SWCNT networks, as discussed later. Figure 1: Pulsed-alternating-voltage induced allotropic transformation of SWCNTs. ( a ) SEM image of an assembled SWCNT network integrated with electrodes fabricated on a specially designed TEM grid (see Supplementary Fig. 1a ). A scale bar is 500 nm. ( b ) Typical I – V characteristics of a pristine SWCNT network device showing breakdown behaviour beyond the voltage, V b =2.7 V, corresponding to a maximum current density of about 4.3 × 10 7 A cm −2 . ( c ) Time-dependent alternating voltage pulses that were used to obtain the described transformation of the SWCNT arrays. V a , t on and t off indicate applied voltage amplitude, and voltage ON and OFF durations, respectively. ( d ) Typical TEM image of the SWCNTs in the array before the voltage cycling was initiated. ( e – i ) Typical morphologies of nanocarbon structures obtained after the voltage pulse cycling was completed. In each case, V a is presented in units V b . The typical carbon morphologies obtained after cycling 3,000 times at V a =0.6 V b are ( e ) SWCNTs with a larger diameter, ( f ) multi-walled tubular structures with several incomplete sp 2 walls, ( g ) well-formed MWCNTs and ( h ) bundles of MWCNTs. ( i ) MGNRs were obtained typically after the network was subjected to 3,000 cycles of V a =0.8 V b . Scale bars in ( d – i ) are all 5 nm. Full size image Allotropic transformations of carbon nanostructures Figure 1d shows a typical TEM image of the pristine SWCNT network (that is, before electrical treatment) comprising of individual and bundles of SWCNTs. Figure 1e–i shows TEM images outlining representative results after the cycling steps were completed using different values of V a . Two different regimes were observed as the V a is increased; one is from 0 to 0.4 V b , where I versus V is linear and in which no significant structural changes occur. The other regime is from 0.4 V b to 0.8 V b , where interesting structural/morphological changes in the nanotube array take place along with active rearrangement of carbon atoms. Three different sp 2 carbon nanostructures are predominantly observed at the applied voltages of 0.6 V b and 0.8 V b . At V a =0.6 V b , we find that a few of the SWCNT bundles coalesce to form few larger diameter SWCNTs, as seen in Fig. 1e . However, under the same conditions, most of the SWCNT networks are transformed either to MWCNT arrays ranging from 15 to 30 nm in diameters with several incomplete sp 2 outer tube walls ( Fig. 1f ; which give rise to either dangling bonds and structural imperfections that may enhance the coalescence of CNTs) [14] , [20] , [25] , [34] , [35] , [36] , [37] or to well-defined MWCNTs with hollow cores and completely formed tube-wall (as straight lattice fringes in Fig. 1g,h ). For V a =0.8 V b , multi-layered and flattened graphitic structures were most commonly observed ( Fig. 1i ), which most probably results when larger-diameters single- or few-walled nanotubes gain stability by collapsing into MGNRs. These results represent the typical observations from over 500 different devices tested for scientific exactitude (see more examples in Supplementary Fig. 2 ). The large-scale uniform transformation across the entire SWCNT networks implies that during the transformation process, the organized arrangement of individual nanotubes was similar across the entire network. This is partially because individual nanotubes were aligned into narrow (approximately few nanometre) bundles because of coherent capillary forces they undergo during the fluidic assembly process [30] . Further, during the initial cycles of voltage-pulsing, randomly oriented SWCNT bundles were observed to form larger (approximately tens of nanometres) and more stable and aligned bundle configurations. A narrow adjacent distance between nanotubes often promotes the hexagonal lattice packing of SWCNTs into larger bundles and to eventually form a bundled rope. Each pair of nanotubes in this arrangement has almost the same probability of forming a coalescence transformation as the voltage is increased. The dense mechanical alignment of SWCNTs in the initial phase of voltage-pulsing placed each of the nanotubes in intimate contact with its neighbour—a necessary prerequisite for efficient coalescence of the nanotubes. We speculate that most of the energy given to the system for values of V a up to 0.4 V b is used in this ‘stability search’ towards better alignment of the nanotubes with each other and to the enlargement of SWCNT bundles without changing their structure (see Supplementary Fig. 2b ). Beyond this voltage ( V a >0.4 V), the original sp 2 bonds undergo a massive rearrangement, accompanied by the rise of a strong coalescence-induced modes (CIMs) in the Raman spectra, which is a signature precursor for inter-tube coalescence [13] , [38] , [39] , [40] , details of which is discussed next. Raman spectra of transformed carbon structures To further investigate the sp 2 junction formation and molecular structure evolution in SWCNT networks, resonant Raman spectroscopy measurements were performed at the same location in the SWCNT network before and after subjecting the sample to the various voltages from 0.2 V b to 0.8 V b ( Supplementary Fig. 3 ). Shown in Fig. 2a are overall Raman spectra showing four representative Raman features: the radial breathing mode ( Supplementary Fig. 7 ), the D-band, the G-band and the G′-band, each representing unique spectral evolutions (not previously observed) as the applied voltage is increased. In the same figure, the expected location of a fifth and extremely interesting emergent feature, the CIM [13] , [38] , [39] , [40] , has been demarcated using a dashed rectangle. The CIM is a unique identifier of vibrations of linear carbon chains ‘H-C n -H’, and depending on ‘ n ’, the length of the chain is expected to result in Raman modes around ω CIM =1,850–1,900 cm −1 . The CIMs provide a very clear confirmation that carbon atoms in the nanotube lattice are moving/migrating to form different sp 2 carbon structures that are mediated via the temporary appearance of junctions in the form of these linear C-chains between adjacent nanotubes [13] , [38] , [39] , [40] as shown schematically in the inset of Fig. 2a . These modes have been determined to be a crucial precursor to the coalescence process in high-temperature-induced coalescence of nanotubes [38] . Interestingly, for our voltage-pulse-induced coalescence, the CIM modes are more prevalent when the pulse duty-cycle ( t on /( t on + t off )) is smaller. This fact is illustrated in Fig. 2b which shows typical Raman spectra near the CIM mode for samples that have been cycled using different ‘on times’, t on (keeping t off constant at 400 ms). As t on decreases, CIM modes (demarcated by arrows in Fig. 2b ) begin to appear at t on =500 ms, being most prominent at t on =100 ms. The disappearance of CIM modes for larger t on values seem to imply that rapid switching of the voltage-pulse is a more effective method to obtain the transformations. Selecting t on =100 ms, we have systematically studied the evolution of CIM peak in a large number of samples subjected to different V a at various cycling stages. As the voltage cycling proceeds, the CIM modes were found to appear and often disappear (see Supplementary Figs 4 and 5 ) in most samples, which is consistent with the fact that the linear carbon chains are intermediate steps during the transformation of SWCNTs into more complex structures. At V a =0.8 V b , the CIM peaks were found to be present even after 3,000 cycles implying that at this high voltage, the transformations were much more large-scale, and within our experimental cycling-range, partially complete. This very typical observation has been illustrated in Fig. 2c , which shows that at the end of the 3,000 cycles, a prominent CIM remains around ω CIM =1,855 cm −1 for samples cycled at V a =0.8 V b . The appearance of the CIM mode is well correlated with our detailed TEM-based inspection of the samples that have been cycled at various values of V a . For samples cycled at 0.4 V b ( Supplementary Fig. 4a ) and below, where the CIM never shows up, we observe no major structural changes in TEM images. When cycled at 0.6 V b , which results in various MWCNT morphologies ( Fig. 1e–h ), the CIM spectral feature appears intermittently at different cycling stages, for example, at 600 and 2,500 cycles for the sample shown in Supplementary Fig. 4b . However, at 0.8 V b , where a highly active structural transformation occurs, the CIM appears consistently throughout the entire cycling stage, as shown in Fig. 2d (see more in Supplementary Fig. 5 ). A clear trend of the rate of structural transformations emerges when the CIM peak intensity I CIM is plotted as a function of cycles, as seen in Fig. 2e . I CIM grows steadily with increased voltage cycling, and exhibits a clear peak, at ~1,500 cycles beyond which the rate of structural transformations gradually slows down, indicating that the structural transitions were largely complete. Hence, this cycle dependence along with the t on dependence enables us to identify the most effective electrical conditions for transforming SWCNT networks into the various sp 2 nanostructure SWCNT networks that occur from 0.5 V b to 0.8 V b voltages. In addition to the CIM, we have also investigated the evolution of the G′-band of the nanotubes before and after voltage cycling. 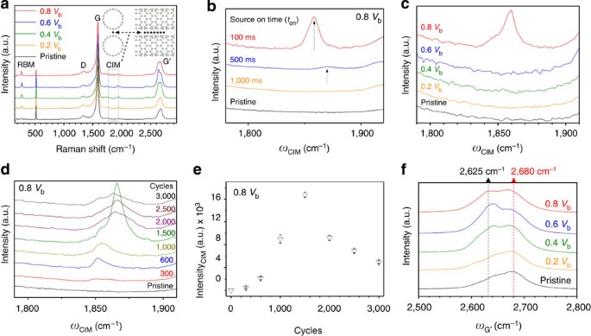Figure 2: Evidence of coalescence and transformations through Raman spectroscopy. (a) Raman spectra of pristine SWCNTs and those transformed by 3,000 cycles of different pulse-amplitudesVa, as noted. The signature peaks (radial breathing mode, G, D and G′) of SWCNTs are labelled. At low duty cycles (that is, smaller values ofton/(ton+toff)), a coalescence-induced mode (CIM, demarcated by arrows) was found to emerge in the Raman spectra, as seen here and more prominently inbfor a sample cycled atVa=0.8Vb.toff=400 ms in all cases. (c) After 3,000 cycles, the CIM was found most consistently in samples cycled atVa=0.8Vb, as shown. (d) Evolution of the CIM peak as a function of number of cycles. (e) Variation of the CIM peak intensity as a function of number of cycles. The peak maximizes around 1,500 cycles indicating maximum SWCNT transformations occurring mid-way of the total 3,000 cycles. Error bars represent the s.d. (f) Evolution of the G′ band for samples cycled at various values ofVa. A low-frequency peak atω=2,625 cm−1emerges after voltage cycling of SWCNTs, consistent with the appearance of large-diameter single- or multi-walled nanotubes. All spectra were measured with a 532 nm laser line (2.33 eV). Figure 2f shows the line-shape and intensity change in the G′-band spectra after electrical treatment with different applied voltages. The average peak position of the G′-band is known to red-shift to lower frequencies with increasing mean nanotube diameter as, (ref. 41 ). In addition to the pristine G′ peak with a maximum around 2,680 cm −1 , we find the clear emergence of a red-shifted peak centred around 2,625 cm −1 after voltage cycling, consistent with the coalescence of small diameter SWCNTs, which forms bigger diameter SWNTs/MWNTs, and the collapse of MWCNTs into their layer-stacked MGNR counterparts. Figure 2: Evidence of coalescence and transformations through Raman spectroscopy. ( a ) Raman spectra of pristine SWCNTs and those transformed by 3,000 cycles of different pulse-amplitudes V a , as noted. The signature peaks (radial breathing mode, G, D and G′) of SWCNTs are labelled. At low duty cycles (that is, smaller values of t on /( t on + t off )), a coalescence-induced mode (CIM, demarcated by arrows) was found to emerge in the Raman spectra, as seen here and more prominently in b for a sample cycled at V a =0.8 V b . t off =400 ms in all cases. ( c ) After 3,000 cycles, the CIM was found most consistently in samples cycled at V a =0.8 V b , as shown. ( d ) Evolution of the CIM peak as a function of number of cycles. ( e ) Variation of the CIM peak intensity as a function of number of cycles. The peak maximizes around 1,500 cycles indicating maximum SWCNT transformations occurring mid-way of the total 3,000 cycles. Error bars represent the s.d. ( f ) Evolution of the G′ band for samples cycled at various values of V a . A low-frequency peak at ω =2,625 cm −1 emerges after voltage cycling of SWCNTs, consistent with the appearance of large-diameter single- or multi-walled nanotubes. All spectra were measured with a 532 nm laser line (2.33 eV). Full size image Electrical and thermal properties In-situ two-terminal electrical resistance changes in SWCNT devices were also measured during the entire transformational process, as such data are indicative of successful junction formation and structural evolution. Our analyses (see Supplementary Fig. 8 ) show that contact resistances play only a small role in the overall changes. 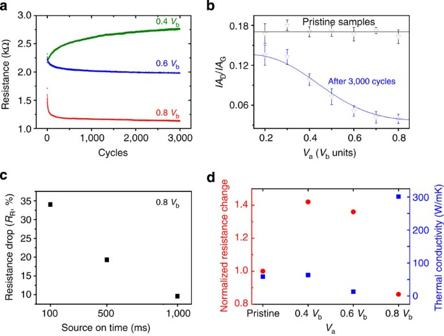Figure 3: The electrical and thermal properties. (a)In-situtwo-terminal electrical resistance of the SWCNT devices as a function of voltage-pulse-cycling at differentVavalues, as noted. (b) The ratio of the integrated area under the D and G band (IAD/IAG) for a range of appliedVavalues, obtained from Raman spectroscopy before and at the end of 3,000 cycles. This ratio is a measure of disorder density in SWCNTs, which is found to systematically decrease asVais increased. Error bars represent the s.d. (c) Percentage device resistance drop,RR=(Rbefore−Rafter) × 100/Rbeforeafter voltage-pulse-cycling is applied atVa=0.8Vb,for varioustonvalues. Interestingly, a larger decrease of device resistance was found when the duty-cycle (that is,ton) is the smallest, consistent with the data inFig. 2b. (d) Variation in normalized resistance changeR(after subtracting the contact resistance, seeSupplementary Fig. 8) and thermal conductivity (calculated based on equation (5) andSupplementary Fig. 9). Figure 3a shows the resistance change as a function of the number of cycles at alternating voltage-pulses of 0.4 V b , 0.6 V b and 0.8 V b , respectively. For samples cycled at V a =0.4 V b , the electrical resistance is seen to increase slowly over time over the entire cycling period. Since neither TEM nor Raman investigations indicated any structural transformations at this V a value, and analysis of the D-band of Raman spectrum ( Fig. 3b ) showed a decrease in defect density, we conjecture that at this voltage, the nanotubes may have been undergoing small mechanical alignment changes that altered the conductive pathways. With increasing V a , however, there was a complete trend-reversal, with the overall resistance decreasing with increasing voltage cycles, commensurate with the increasing inter-nanotube junction formation, as well as significant increase in diameter and wall-thickness of the conductive structures. The decreasing electrical resistance because of voltage cycling is also highly consistent with the steady decrease of defect density in the structures after voltage cycling was completed. This fact is brought out in Fig. 3b , which shows the variation of IA D / IA G (ratio of the integrated areas of the D and G bands) as a function of V b . The results clearly show a sizeable decrease in IA D / IA G with increasing V a , indicating that the network is getting relatively less defective (relative decrease of D-band intensity) and more organized by forming more ordered sp 2 carbon nanostructures (relative increase of G-band) after the transformational process. Figure 3: The electrical and thermal properties. ( a ) In-situ two-terminal electrical resistance of the SWCNT devices as a function of voltage-pulse-cycling at different V a values, as noted. ( b ) The ratio of the integrated area under the D and G band ( IA D / IA G ) for a range of applied V a values, obtained from Raman spectroscopy before and at the end of 3,000 cycles. This ratio is a measure of disorder density in SWCNTs, which is found to systematically decrease as V a is increased. Error bars represent the s.d. ( c ) Percentage device resistance drop, R R =( R before − R after ) × 100/ R before after voltage-pulse-cycling is applied at V a =0.8 V b, for various t on values. Interestingly, a larger decrease of device resistance was found when the duty-cycle (that is, t on ) is the smallest, consistent with the data in Fig. 2b . ( d ) Variation in normalized resistance change R (after subtracting the contact resistance, see Supplementary Fig. 8 ) and thermal conductivity (calculated based on equation (5) and Supplementary Fig. 9 ). Full size image Figure 3c shows the percentage drop in post-cycling resistance as a function of t on in a sample cycled 3,000 times with V a =0.8 V. Interestingly, the electrical resistance drop was found to be largest when the duty-cycle was smallest, which is in direct agreement with the t on -dependent appearance of the CIMs ( Fig. 2b ), suggesting that rapid pulse-switching (when t on is small) rather than prolonged Joule-heating (when t on is large) better assists in the transformation processes. Figure 3d shows the variation of the electrical resistance and thermal conductivity in SWCNT networks as a function of V a (contact effects were removed using methods described in Method section). Particularly, when V a =0.8 V b is applied for 3,000 cycles, both the electrical contact resistance (metal electrodes-SWCNTs)and intrinsic network resistance (see Supplementary Fig. 8 ) decrease because of the formation of electrically stable metal–nanotube interfaces and restructured sp 2 nanocarbon networks. At the same time, the post-cycling thermal conductivity was found to gradually decrease from ~60 W mK −1 to ~10 W mK −1 up to V a =0.6 V b . For V a =0.8 V b , however, there was a dramatic increase in thermal conductivity, reaching values of ~300 W mK −1 , which is five times higher than that of pristine SWCNT networks. The sharp drop in the network electrical resistance and dramatic increase in its thermal conductivity when voltage-pulse cycled at V a =0.8 V b is accompanied by a rather unexpected finding—the possible appearance of sp 3 -hybridized carbon in the network. 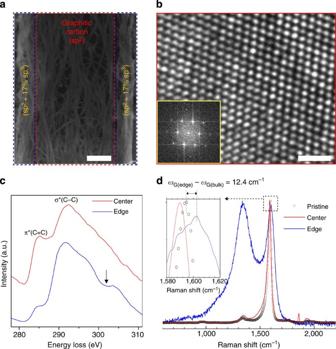Figure 4: Possible emergence of −sp3carbon atVa=0.8Vb. (a) An SEM image of the transformed nanocarbon array after the electrical treatment at 0.8Vbwith 3,000 cycles. (d) High-magnification TEM images showing a lattice structure whose spacing is consistent with −sp2carbon (see text), obtained from the centre-region of network. The inset figure ofbshows the corresponding fast Fourier transform (FFT) pattern. (c) The carbon K-edge energy loss spectrum (EELS) obtained from the centre (red solid) and the edge (blue solid) of the sample as shown ina. Signatures of C=C π* bonds at the edge is reduced significantly, whereas a clear signature of −sp3carbon appears in the spectrum (shown with an arrow, see text). The percentage of these −sp3bonds could be obtained by comparing the Raman spectra of (d) the pristine samples (black circles), the central region of the voltage-pulse-cycled samples (red solid) and the edges of the same array (blue solid). The inset is the Raman spectra zoomed into the G-band range, which shows a red-shift in the central region consistent with the formation of multi-layered graphitic sp2structures, and a blue shift of 12.4 cm−1at the edges, which corresponds to the ~17% of sp3carbon structures (see text). Scale bars in (a), 200 nm; in (b), 1 nm. sp 2 –sp 3 hybrid nanostructures Figure 4a shows an SEM image of the network structure after being cycled at 0.8 V b . High-resolution TEM image of the central portion of this structure ( Fig. 4b ) reveals that the transformed network consists of a multi-layered graphitic sp 2 structure. The measured in-plane lattice spacing in the centre is 0.24±0.02 nm, which is identical to the sp 2 carbon structure [24] . This observation is consistent with all our previous findings. However, carbon K-edge energy loss spectrum (EELS) and resonant Raman spectroscopy results that compare the central region versus the edges of these networks reveal that at the edges the network is transformed to sp 2 –sp 3 hybrid nanostructures. In Fig. 4c , we compare the EELS spectra from the centre (red) and the edge (blue) regions of the sample shown in Fig. 4a . In general, sp 2 bonds exhibit a peak around 290 eV because of σ * states and the other peak appears at 285 eV corresponding to π * states [42] , [43] , [44] , as seen in the spectrum measured from the centre of the sample. However, the EELS spectrum measured at the edges shows clear signatures of sp 3 -type carbon: a σ * edge around 290 eV corresponding to the sp 3 transition 1s→2σ* (ref. 45 ) and a dip around 302 eV that corresponds to the second absolute band gap characteristic of the crystalline sp 3 structure [46] , [47] . Further, the sp 2 carbon band at ~285 eV becomes a very shallow shoulder in the spectrum of the sp 3 -bonded carbon. We have used the relative G-band shift in Raman spectra focused on two different locations, centre and edges of the transformed network ( Fig. 4d ), to estimate the percentage abundance of −sp 3 carbon. The Raman spectra, taken at the centre of networks, zoomed into the G-band range (inset in Fig. 4d ) indicate that this transformed network keeps mostly crystalline sp 2 bonds. However, at the edges, Raman spectrum shows the characteristics of a nano-crystallization of the pristine material with highly disordered sp 2 bonds (amorphization) and the rise of some sp 3 bonds. The contents of sp 3 bonds (in %) at the edges can be calculated with the relation [48] sp 3 (%)=0.24–0.0049*( ω G(edge) − ω G(centre) ), in which ω G(edge) =1,602.4 cm −1 and ω G(centre) =1,590 cm −1 stand for the G-mode Raman frequency at the edges and in the centre of the resultant material. According to this expression, there are about 17% of sp 3 bonds at the edges (as annotated in Fig. 4a ). As shown in the Fig. 4a , nanotubes in both edges are more highly aligned because of the capillary force-induced assembly of SWCNTs [30] , [32] . Highly excited electrons for V a =0.8 V b constantly transfer their energy to the nanotube lattice. Especially for the highly aligned SWCNT arrays at the edges of the network, a more effective rearrangement of carbon atoms can potentially occur along the compact and aligned nanotube lattices, leading to the possible formation of the sp 3 structures. Therefore, it is assumed that reduced junction scattering and increased thermal conduction pathway through the sp 3 carbon structure might cause the previously discussed high thermal conductivity in this network. Figure 4: Possible emergence of −sp 3 carbon at V a =0.8 V b . ( a ) An SEM image of the transformed nanocarbon array after the electrical treatment at 0.8 V b with 3,000 cycles. ( d ) High-magnification TEM images showing a lattice structure whose spacing is consistent with −sp 2 carbon (see text), obtained from the centre-region of network. The inset figure of b shows the corresponding fast Fourier transform (FFT) pattern. ( c ) The carbon K-edge energy loss spectrum (EELS) obtained from the centre (red solid) and the edge (blue solid) of the sample as shown in a . Signatures of C=C π* bonds at the edge is reduced significantly, whereas a clear signature of −sp 3 carbon appears in the spectrum (shown with an arrow, see text). The percentage of these −sp 3 bonds could be obtained by comparing the Raman spectra of ( d ) the pristine samples (black circles), the central region of the voltage-pulse-cycled samples (red solid) and the edges of the same array (blue solid). The inset is the Raman spectra zoomed into the G-band range, which shows a red-shift in the central region consistent with the formation of multi-layered graphitic sp 2 structures, and a blue shift of 12.4 cm −1 at the edges, which corresponds to the ~17% of sp 3 carbon structures (see text). Scale bars in ( a ), 200 nm; in ( b ), 1 nm. Full size image The exact mechanism at the atomic-scale that initiates the C–C bond reconfigurations is not yet clear to us at this point. However, a few relevant mechanisms are important to discuss. First, the instantaneous local temperature of the SWCNTs because of periodic voltage-pulse cycling could reach up to 1,200 K at V a =0.8 V b (see Method section), and thermally induced changes in −sp 2 carbon structures are usually negligible at such temperatures [28] . Moreover, the transformations are more effective under rapid voltage-switching (smaller values of t on ) rather than higher heat-generating (larger values of t on ) cycles. This indicates that Joule heating alone is not sufficient to explain the transformation process. Second, the formation of bundles and the resulting densification of SWCNTs at the initial stages of cycling indicate that the applied voltage-pulses induce coherent mechanical forces that move nanotubes closer to each other. However, although these forces can move the nanotubes into intimate proximity, they alone are not likely to trigger the entire coalescence phenomenon. A third factor is the role of electromigration in triggering the transformations [24] , [25] , [49] . At high current densities, electrons can transfer significant momentum to atoms causing them to migrate from their parent sites, and such migration events rapidly grow in number at elevated temperatures (such as in our case). However, the effectiveness of electromigration alone in driving the entire sequence of transformations is difficult to quantify. We believe that a combination of all these above effects may be playing a role in bringing about the allotropic transformations. We speculate that the nanoscale forces that initially align the nanotubes bring them to van der Waals proximities. Thermal fluctuations and electromigration may cause these atoms to move out of their lattice sites, and these mobile atoms minimize their energies by forming linear chains between two SWNCTs ( Fig. 2a ) that forms a junction between nanotubes and give rise to the CIMs in Raman spectroscopy. With continued cycling, the junction grows wider and eventually becomes comparable in size with the nanotube diameters and the nanotubes release mechanical strain by coalescing into larger-diameter structures. Very likely, in-situ high-resolution TEM studies and atomistic simulations may be necessary for a better understanding of the overall transformation process steps. In summary, we are able to transform SWCNT networks to other predetermined sp 2 carbon nanostructures (SWCNTs with a larger diameter, MWNTs or MGNRs) by controlling the electrical parameters, such as alternating voltage-pulse magnitudes, source-on-time and the number of switching cycles applied to the CNT networks. To our knowledge, this is the first demonstration of atomic-level engineering of molecular junctions and controlled structural transformations in CNT networks without increasing structural defects. The applied voltage, periodic polarity change and associated electrical force activate a coalescence-induced reconfiguration of sp 2 hybridizion. The method can be facile and easily scalable, which will allow us to tailor the desired molecular structure and physical properties of nanocarbon networks for applications, such as electronic devices, energy storage systems and multifunctional membranes and fibres. Fabrication of highly aligned SWCNTs The basic steps for building organized SWCNT lateral architectures fabricated using the template-guided fluidic assembly process [30] , [31] , [32] , are as follows. First, a 300-nm-thick polymethyl methacrylate photoresist is deposited on a substrate and baked at 160 °C for 90 s. Second, polymethyl methacrylate patterns are constructed on the substrate using electron-beam lithography to build nanoscale channels, which form templates for building the test architectures and these templates are then developed in the solution (methyl isobutyl ketone/isopropyl alcohol=1:3) for 100 s followed by a 30-s rinse in isopropyl alcohol solution. Next, these template substrates are dip-coated in a 0.23 wt% high-purified SWCNT solution ( Supplementary Table 1 and Supplementary Notes ) at a constant pulling rate of 0.1 mm min −1 . The dip-coating processes result in stable and densely aligned SWCNT lateral network architectures on the substrate having well-defined shapes at the nanoscale. Finally, the photoresist is removed to obtain well-organized and aligned SWCNT lateral networks. For the fabrication of contact electrodes consisting of Ti(5 nm)/Au(150 nm), the same fabrication steps are applied except for a dip-coating process described above. CNTs density in the network array The networks made from dip-coating techniques typically have the smallest surface roughness and close-packing structures with 80% dense CNTs (based on Supplementary Fig. 1d,e ). The cross-sectional area is approximately 18,000 nm 2 ±3,000 nm 2 (based on Supplementary Fig. 1c,f ). Therefore, the number of CNTs in the network of 2 μm 2 dimension is calculated as about (4±0.5) × 10 4 ((2±0.25) × 10 12 cm −2 ). Transformation processes of SWCNT arrays A Keithley 2,400 sourcemeter was used to apply voltage and to measure the resistance across the two terminal CNT devices. All the measurements were done under high vacuum ( P <10 −5 Torr) in a Janis Research ST-500 cryogenic probe station to reduce radial heat losses through gas convection and to avoid burning the devices. Voltage sweeps were applied through CNT arrays to find the breakdown voltage. Most of the CNT arrays failed at a maximum current density of about 4.3 × 10 7 A cm −2 , and the breakdown voltage ( V b ) was 2.7 V on the TEM window ( Fig. 1b ). By sweeping the voltage over a suitable range, we observe a critical voltage for which the graphitization process is speeded up. At the same time, applied voltages too close to V b often leads to the breakdown of the nanotube ( Supplementary Fig. 6 ). Therefore, V b for these quasi-parallel SWCNT networks was found to be an important characterization parameter. The V b in our device could be predicted statistically by V b =−2.14 × I 1V +9.13, here I 1V [mA] is a current at 1 V. Arrays with a nearly similar current density were used for testing the reproducibility of the transformation process. For the structural engineering of the CNT arrays, repetitive positive and negative voltages of 0.4 V b , 0.6 V b and 0.8 V b , which the electrical powers were in the range of 2–3, 6–8 and 10–15 mW, respectively, under our device condition (for SiO 2 /Si substrate, see Supplementary Fig. 1g and Supplementary Methods ), were each applied at 1 Hz for 3,000 cycles at 180 °C (453 K) between the two electrodes on the CNT arrays. Although the external temperature is too low to promote any C–C bond rearrangement, this temperature showed a better effect than room temperature (300 K) for the engineering of the SWCNT arrays into new nanostructures. A higher external temperature caused wall defects and damage to the SWCNT arrays under each applied voltage. After transformation processes of SWCNT arrays, the devices were cooled slowly to prevent fracture due to the rapid cooling. Temperature by electrical energy Breakdown occurs when the maximum temperature of the tube reaches the value of the breakdown temperature, which allows the extraction of a simple expression for the breakdown voltage of SWCNTs, including heat generation from Joule self-heating and heat loss to the substrate [50] , [51] . Therefore, the maximum temperature at the breakdown voltage is explained as: Here, T BD is the maximum temperature, P BD is the breakdown power, the combined resistance of the source and drain contacts, R C is estimated from the inverse slope of the low-bias I D −V SD plot, R C ≈(d I D /d V SD ) − 1 , g is the heat dissipation coefficient in the substrate per unit length and L is length of CNT network. From the equation, the calculated maximum temperature is about 1,335 K (1,062 °C). At the 0.8 V b , the temperature is calculated as about 1,200 K. SEM and TEM observation The CNT arrays were prepared on specially designed chips with a window of 40 × 40 μm 2 for SEM and TEM imaging. The CNT arrays were suspended on an electron transparent window by employing a two-probe device architecture. Two micro-heater electrodes of 10 μm in width were employed around the arrays on the chip for the external heating. The TEM measurements were carried out in a JEOL-3011 high-resolution TEM instrument using an accelerating voltage of 300 kV. The allotropes cover a significant area of the devices, which was verified by taking TEM images at different positions over the sample. Raman measurements Raman spectroscopy (LabRAM HR 800, HORIBA Jobin Yvon, HORIBA) was used to investigate structure changes of CNT arrays as the applied voltage and the numbers of cycles were changed. The laser excitation wavelengths used were 532 nm (2.33 eV) and 633 nm (1.92 eV), the exposure time was 5 s per spectrum, and the number of data accumulations was 10. A 600 lines per mm grating was used, and the confocal hole diameter was set to 100 μm ( Supplementary Notes ). Electrical resistance measurements To obtain a reasonable estimate of the contact resistance, four equally spaced identical electrodes were fabricated using a magnetron sputter-coater. The estimation used for the interfacial contact resistance assumes that the two-terminal resistance between any two electrodes is the sum of the device resistance of the CNT arrays and the interfacial contact resistance at each contact [52] . From the two-terminal I–V characteristics, the resistance R was measured in all test structures, which have a lateral width of 1 μm. The four contact pads were separated by a distance of 2 μm from each other. I–V measurements were conducted between the pairs of contacts A–B, B–C, C–D, A–C and B–D. The contact resistance at contact pad B and C ( R c B and R c C ) can be written as where R AB = R c A + R d AB + R c B , R BC = R c B + R d BC + R c C , R AC = R c A + R d AC + R c C , R CD = R c C + R d CD + R c D and R BD = R c B + R d BD + R c D . The resistance R d BC is defined as a device resistance between a contact pad B and C ( Supplementary Fig. 8a ). Therefore, the two contact resistances and the resistances of the CNT array itself were all calculated from data taken on five pairs of device resistances and the values were compared before and after the CNT array treatment ( Supplementary Fig. 8b–d ). Thermal conductivity measurements The measurement of thermal conductivity was performed by using a self-heating 3 ω technique [53] , [54] . The 3 ω signal correlates with the thermal conductivity through the following equation [53] , [54] , where L, R and S are the distance between the contacts, the electrical resistance and the cross-sectional area of the sample, respectively. R ′ =(δR/δT) is the temperature gradient of the resistance at the chosen temperature and k is the thermal conductivity. The 3 ω method was used by the four-point-probe third harmonic characterization method to eliminate the contact resistance and to avoid related spurious signals. The 3 ω signals can be used for measuring the thermal conductivity of the SWCNT arrays. A lock-in amplifier (Stanford Research System SR850) was used for obtaining the 3 ω signals by amplifying the small voltage and removing the noise. An AC current source (Keithley 6221) was used to provide a stable current supply. All the measurements including the resistance, temperature and 3 ω signals were done under high vacuum ( P <10 −5 Torr) in a Janis Research ST-500 cryogenic probe station to reduce radial heat losses through gas convection. The temperature coefficient of the resistance should be measured in order to obtain the thermal conductivity based on equation 5. The resistance-temperature coefficient of the CNT arrays themselves was also measured over the small temperature range of 296–300 K, which is close to the measurement temperature of the 3 ω signal (see Supplementary Fig. 9 ). The resistance change of the pristine SWCNTs as a function of temperature was about 53.7 Ω K −1 . Those of the samples treated at 0.4 V b and 0.6 V b showed a negative resistance temperature ( R(T) ) value of −26.2 Ω K −1 and −9.03 Ω K −1 , respectively. On the other hand, R(T) showed a positive value of 1.6 Ω K −1 for the sample treated at 0.8 V b . The third-harmonic voltage measured at the frequency of 1,000 Hz is shown in Supplementary Fig. 9 . By fitting these results according to equation (5), the exponent of the current amplitude I 0 was found to be 2.8–3.1 for the samples. These values are very close to the third power predicted from theory. The calculated thermal conductivities were 58.5, 63.5, 13.1 and 301.2 W mK −1 for the pristine SWCNTs, and samples treated at 0.4 V b , 0.6 V b and 0.8 V b , respectively ( Fig. 3d ). We assume that the factor of five increase of the effective thermal conductivity in the array treated at 0.8 V b is caused by the highly reduced junction scattering and the thermal pathways to sp 3 structures. How to cite this article : Jung, H. Y. et al . Sculpting carbon bonds for allotropic transformation through solid-state re-engineering of –sp 2 carbon. Nat. Commun. 5:4941 doi: 10.1038/ncomms5941 (2014).